Selective contacts drive charge extraction in quantum dot solids via asymmetry in carrier transfer kinetics Colloidal quantum dot solar cells achieve spectrally selective optical absorption in a thin layer of solution-processed, size-effect tuned, nanoparticles. The best devices built to date have relied heavily on drift-based transport due to the action of an electric field in a depletion region that extends throughout the thickness of the quantum dot layer. Here we study for the first time the behaviour of the best-performing class of colloidal quantum dot films in the absence of an electric field, by screening using an electrolyte. We find that the action of selective contacts on photovoltage sign and amplitude can be retained, implying that the contacts operate by kinetic preferences of charge transfer for either electrons or holes. We develop a theoretical model to explain these experimental findings. The work is the first to present a switch in the photovoltage in colloidal quantum dot solar cells by purposefully formed selective contacts, opening the way to new strategies in the engineering of colloidal quantum dot solar cells. Solution-processed photovoltaic cells have attracted growing research and technological interest in view of their potential to enable low-cost, large-scale solar energy conversion [1] . Among the different classes of solution-processed solar cells, including dye-sensitized and organic solar cells, rapid progress has been achieved recently for solar cells made using colloidal quantum dots (CQD). In CQD solar cells, a thin film a few hundred nanometers thick is formed with the aid of bidentate organic linkers, which serve to bring the nanoparticles into close packing while achieving the best available surface passivation [2] , [3] . In CQD solar cells, the resultant CQD solid simultaneously carries out the functions of light absorption, charge separation and charge carrier transport. All-solid CQD solar cells have demonstrated 7% solar power conversion efficiency certified by an independent laboratory [4] . This rapid technological progress, combined with scientific interest in elaborating a more comprehensive model of device operation, motivates the investigations in this work. Specifically, we sought to study the role of contacts in determining the photovoltage—a critically important parameter in any solar cell. First, though, we briefly review the formation of the CQD solid. The successful operation of CQDs in an efficient solar cell is strongly dependent on the material-processing strategies used in film formation. When CQD are synthesized in solution, they are usually capped by organic molecules that employ long chains (8–18 carbons) to avoid agglomeration. Optimum photovoltaic operation of the CQD film requires the replacement of such ligands with short organic bidentate linkers, such as ethanedithiol or mercaptopropionic acid (MPA). This produces [5] film densification; reduction of the interparticle separation to less than the carrier tunneling distance, consequently enhancing the QD–QD coupling and carrier transport; and passivation of the surface states to reduce recombination losses. Of particular relevance among these features is the reduction of interdot distance to facilitate exciton dissociation and separate carrier transport towards the collecting contacts. Progress in the application of short organic ligands together with the use of QDs harvesting infrared photons were key advances leading to the >7% power conversion efficiency in CQD solar cells [4] , [6] . Another crucial aspect for the effective operation of this type of solar cells is the formation of contacts that determine the overall device structure. Usually a metal oxide is adopted as electron extraction contact and a high work function metal as hole extraction material [7] . Interfacial engineering to obtain efficient electrical contacts is a central effort of the field [8] . It has been recognized that contacts determine device operation for CQD films used in applications of solar cells as well as photodetectors, which has led to the investigation of different materials such as MoO 3 hole-selective layers, organic and nanostructured contact materials [9] , [10] , [11] , [12] , [13] . In principle, for solar cells that benefit from a sufficiently short dielectric relaxation time, there are two main mechanisms of charge extraction [14] . One is charge separation followed by drift through a depletion layer that is formed at a contact–semiconductor interface or a p-n junction. Appreciable photocurrent can be generated directly in the depletion layer if its thickness exceeds the characteristic light absorption length. The depletion layer thickness w contains an electrical field that accelerates carriers and facilitates their collection at the separate contacts. To date, drift has been the principal means by which CQD solar cells have extracted their photocurrents [2] , [3] , [15] , [16] . Typical CQD films are doped to an extent N D ≈10 16 −10 18 cm −3 , usually p-type [5] , [13] , although n-type active layer devices have recently been achieved [17] . The second mechanism is that the carriers diffuse, without reliance on any appreciable built-in electric field, from their point of generation. The diffusion length L n describes the average distance over which a charge carrier can diffuse before it recombines. Today, CQD solar cells rely on a combination of drift and diffusion. It would be very desirable for diffusion to have a larger role, that is, for L n to be increased, via engineering of the transport and recombination properties of the quantum dot solid, to be much larger than the 30- to 100-nm length it is estimated at today. Solar cells that rely heavily on drift in the depletion region generally suffer a low fill factor, as when the device reaches its maximum power point, it is much less depleted than at its short-current current condition (except for very thin QD films). In CQD cells, this is illustrated by the fact that the best fill factors published have been in the range of 50–60%, while the theoretical best-case fill factor for a solar cell operating at 1 sun and having a 1.3 eV bandgap reaches close to 90%. It should also be noted that the fill factor is influenced not only by the presence of an electrical field but also by bulk and surface recombination and by series resistance. Enhancing diffusion—consistent with thicker extraction lengths, lower series resistance and lower recombination—is an avenue to enhancing fill factor in light of all these considerations. Solar cells that rely principally on diffusion are entirely reliant on the formation of selective contacts. These allow the egress of only one type of carrier and block the other one [18] . In summary, as a solar cell requires light absorption combined with asymmetry, it is the deployment of these asymmetrically selective contacts that provides the impetus for asymmetric charge separation. In most cases, dye-sensitized solar cells as well as bulk heterojunction solar cells operate with long diffusion lengths and effective selective contacts [18] , [19] , [20] . Selective and blocking layers are also very useful in organic light-emitting diode (OLED) technologies [21] . In this paper, we therefore consider the question whether CQD photovoltaic devices can operate effectively without reliance on drift as their primary source of photocurrent. A conventional approach to such an investigation would rely on measuring barriers, lifetimes and other electronic materials parameters—none of which is accurately known in today’s CQD devices. We therefore took the view that a fresh approach was required. The electrochemical configuration, shown in the scheme of Fig. 1 , offers a major advantage in a study of the behavior of quasi-neutral CQD solids: in this configuration, all macroscopic electrical fields are removed [22] , [23] . In this measurement, the CQD film is deposited on top of one contact, while the other side of the film is permeated by a redox electrolyte that forms the second contact. The redox electrolyte, combined with the use of auxiliary and reference electrodes, ensures that no net field is applied across the device in its totality [24] , [25] , [26] , [27] , [28] , [29] . 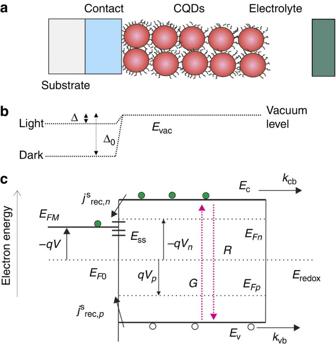Figure 1: Schemes of prepared samples and theoretical model. (a) Scheme of a layer of colloidal quantum dots joined by organic linkers on top of a conducting substrate and immersed in an electrolyte. (b) Energy diagram showing the vacuum level in the dark and under illumination, electron and hole energy levels and Fermi levels, and the substrate energy level. The processes of generation, recombination and interfacial charge transfer are also indicated. Figure 1: Schemes of prepared samples and theoretical model. ( a ) Scheme of a layer of colloidal quantum dots joined by organic linkers on top of a conducting substrate and immersed in an electrolyte. ( b ) Energy diagram showing the vacuum level in the dark and under illumination, electron and hole energy levels and Fermi levels, and the substrate energy level. The processes of generation, recombination and interfacial charge transfer are also indicated. Full size image We therefore turn to our study of PbS CQD films contacted using a variety of different contact materials of practical interest, measured in a redox electrolyte. Our model for interpretation of data is as follows. Under illumination, the electron and hole quasi-Fermi levels separate. As electrical fields are shielded by the redox electrolyte, there is no spatial asymmetry in the film that makes the contact acquire preferentially carriers of either sign. Device operation becomes governed by the dominance of concentration of one carrier at the contact, as well as that contact’s selectivity, rather than any built-in potentials. In summary, the asymmetry of these devices arises by virtue of interfacial kinetics. The sign of photovoltage V oc in the photoelectrochemical cell depends on the difference between the Fermi level of the contact E Fm and the redox energy of the electrolyte, E redox . where q is elementary charge. Using different contact materials, we can induce a kinetic preference of interfacial charge transfer so that E Fm can follow either electrons or holes Fermi level, controlling the sign of the photovoltage V oc . We find that, as expected, V oc increases with increasing light intensity incident of the CQD film. A general theory of selective contacts kinetics is presented to explain these results. Preparation of QD films PbS CQDs capped with oleic acid were synthesized by the hydrothermal method, described in previous studies [30] . 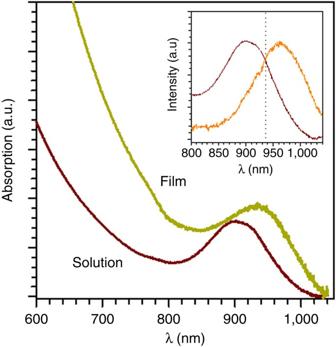Figure 2: Absorption and emission on PbS QDs. Absorption spectra of oleic-capped PbS QDs solution in octane and PbS CQDs film deposited on FTO substrate. The inset shows absorption and emission (orange line) spectra for solution QDs. Energy bandgap estimated from the intersection point of both normalized curves (~936 nm) was 1.3 eV and particle size 3.7 nm. Figure 2 shows the absorption spectrum of PbS CQDs dispersed in octane with the first excitonic peak at ~900 nm. A red shift is observed after CQD deposition in a film, indicating a reduction of the quantum confinement due to the interaction between closely packed CQDs. The CQDs’ energy bandgap, E gap , has been estimated from the intersection point of the normalized absorption and emission spectra (~936 nm, inset of Fig. 2 ). E gap was 1.32 eV and the particle size was 3.7 nm as calculated from Hyun et al . [31] PbS nanocrystals with this particle size have reported the highest efficiencies because of the maximized light harvesting in the IR and the favorable energy alignment with TiO 2 electrodes [30] . Figure 2: Absorption and emission on PbS QDs. Absorption spectra of oleic-capped PbS QDs solution in octane and PbS CQDs film deposited on FTO substrate. The inset shows absorption and emission (orange line) spectra for solution QDs. Energy bandgap estimated from the intersection point of both normalized curves (~936 nm) was 1.3 eV and particle size 3.7 nm. Full size image To study the operation mechanisms of CQDs solid devices, several PbS CQDs films deposited over different contact materials were prepared as depicted in Fig. 1 , including metals, polymers and metal oxide semiconductor materials. The details of preparation methods are given in Methods section. The transparent conductor fluorine-doped tin oxide, either bare or covered with a layer of either Au or poly(3,4-ethylenedioxythiophene) (PEDOT), are expected to form a contact that predominantly equilibrates to holes, while wide bandgap metal oxides TiO 2 and ZnO form a contact that is selective to electrons as indicated in energy schemes in Fig. 3 . For both cases, we estimated the position of the Fermi level from the donor densities given in the literature: N D TiO 2 ≈10 15 –10 16 (ref. 5 ) and N D ZnO ≈10 17 cm −3 (ref. 13 ). 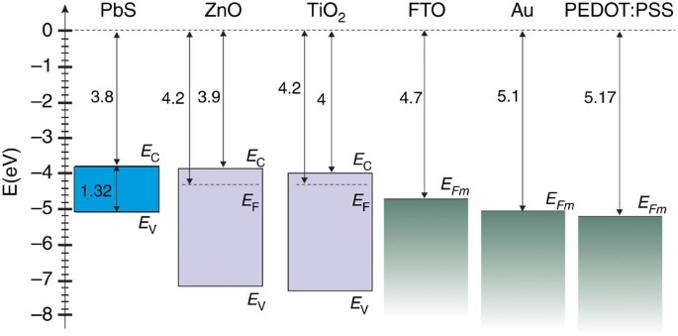Figure 3: Energy levels of PbS QDs and of the different contacts. Energy levels for the different substrates employed in this work and 3.7 nm colloidal PbS quantum dots31,44. Figure 3: Energy levels of PbS QDs and of the different contacts. Energy levels for the different substrates employed in this work and 3.7 nm colloidal PbS quantum dots [31] , [44] . Full size image To deposit PbS CQDs films, oleic acid-capped PbS QDs in octane were spin-coated and then exposed to the cross-linking ligand, MPA, in a solid-state treatment. This process was repeated in a layer-by-layer deposition technique to achieve the desired thickness. The thickness of the PbS film was ~600 nm, determined by scanning electron microscopy ( Supplementary Fig. S2 ). Photoelectrochemical properties of QD films in electrolyte solution Photoelectrochemical measurements were performed to unveil the charge-transfer mechanisms between the QDs film and the contacts. The measurements were carried out in a three-electrode configuration using anhydrous and degassed tetramethylammonium perchlorate (0.1 M) in dimethylformamide as electrolyte, platinum wire as counterelectrode and Ag wire as a quasi-reference electrode. The investigation of QD film charging by applied voltage has been amply reported in the literature through different techniques [24] , [25] , [26] , [27] , [28] , [29] , [32] . We used cyclic voltammetry (CV) both in the dark and under illumination as a tool to study the nature of the contacts in otherwise identical CQD films. 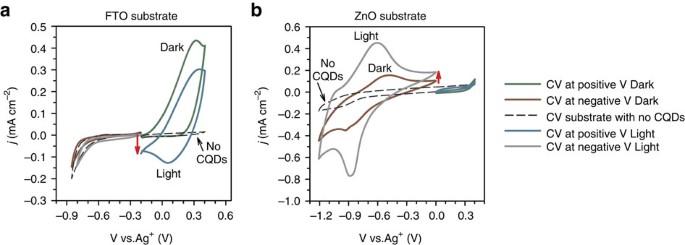Figure 4: Cyclic voltammograms under illumination and dark conditions. (a) Cyclic voltammograms recorded for PbS CQDs films over FTO and (b) ZnO substrates at scan rate of 100 mV s−1, in the dark and under illumination conditions. Comparing with reference samples (bare substrates), the samples with QDs exhibit curves displaying two waves in the charging and discharging directions. Figure 4 shows the cyclic voltammograms for two selected types of contacts, FTO and ZnO. Bare FTO and ZnO substrates without CQD layer were also measured for the sake of comparison. Figure 4: Cyclic voltammograms under illumination and dark conditions. ( a ) Cyclic voltammograms recorded for PbS CQDs films over FTO and ( b ) ZnO substrates at scan rate of 100 mV s −1 , in the dark and under illumination conditions. Comparing with reference samples (bare substrates), the samples with QDs exhibit curves displaying two waves in the charging and discharging directions. Full size image A wide-range potential CV showed a characteristic charging/discharging process clearly differentiated for each electrode based on the polarity of the applied potential ( Supplementary Fig. S3 ). Thus, we have split the CV measurements of the CQD electrodes in these regions and measured them only after allowing the sample to release any amount of charge accumulated during previous measurements. The comparison with the bare substrate electrode provides relevant information to determine if electrons or holes are injected into CQD film. Figure 4a shows that for FTO electrodes, the response of the sample does not change qualitatively with respect to the bare substrate at negative bias. Small observed changes are attributed to small variations in the actual area of FTO in contact with the electrolyte (lower due to the coverage by QD material). The contact between the substrates and the electrolyte allows ions to approach the contact region between PbS and substrate, easing electrical field screening at CQD layer. However, both responses significantly differ at positive potentials. When scanning at positive potential, a wave (peaking at 0.32 V in dark and 0.35 V under illumination) due to oxidation of CQDs film by FTO is clearly observed. This result indicates that the FTO contact matches with valence band (VB) of PbS, assisting a preferential hole-transfer mechanism from the FTO to the PbS. In dark, the film can be charged with holes. Under illumination, the increased conductivity and charge compensation facilitate the recovery of the injected charge in the cathodic run. Conversely, the electrodes based on the ZnO substrate exhibit the opposite trend ( Fig. 4b ). Bare and PbS-coated samples behave very similarly at positive potentials, while the ZnO-PbS electrode presents a near-reversible redox wave both in the dark and under illumination at negative potentials, corresponding to excellent electron uptake and release at the contact. In the cathodic branch, the peak potentials are −0.94 V versus Ag + and −0.89 V versus Ag + in the dark and under illumination, respectively. In the anodic scan, the peak potentials are observed at −0.48 V versus Ag + and −0.6 versus Ag + in the dark and under illumination, respectively. Higher current densities are measured under illumination. These results indicate excellent two-way electron transfer between ZnO substrate and PbS QD, which is enhanced under illumination conditions. Further corroboration of these interpretations is given by the shift in CV curves close to 0 V ( Fig. 4 , red arrows), a phenomenon attributable to the photocurrent. FTO-PbS shows negative photocurrent, while ZnO-PbS exhibits positive photocurrent, indicating the transfer to acceptor/donor species in the electrolyte of the electrons and holes, respectively. The observed photocurrents are very low, as no redox couple (no intentional acceptor or donor species) has been added to the electrolyte, see ‘Methods’ section. From these results, we conclude that the nature of the contact drastically affects the charging properties of the CQD film. For FTO substrates, a large positive current wave is observed at positive potentials, indicating that holes are injected into the film and extracted during the negative current wave. In contrast, for the ZnO contact, a negative current increases at negative potentials indicating that electrons are injected into the film and can be almost reversibly extracted. The observed signs of the photocurrent also corroborate these conclusions. These results suggest that the contact materials are able to capture and equilibrate only one specific type of carrier. A previous demonstration of this effect was reported for thin CdTe QD films [33] It was shown that the directionality of electron and hole separation can be controlled simply by the addition of a single monolayer of CdSe QDs. A reference CdTe sample produces a positive photovoltage signal, while the addition of a single monolayer of CdSe QDs leads to a change in the analyzed signal. Such layers are too thin to form an electric field, thus charge separation has to be kinetically controlled at the interface. Inversion of photovoltage by modification of the contacts To demonstrate how the different properties of photovoltaic behavior of PbS CQD films depend on contact at the substrate, we measured the stable photovoltage of the film immersed in electrolyte as a function of the light intensity, taking as reference the dark voltage value, V dark ( Fig. 5 ). A negative voltage means that the Fermi level of the contact approaches the semiconductor conduction band (CB) as indicated in equation (1). The control of sign of the voltage is here interpreted in terms of preferential exchange of one type of carrier, according to a model that is discussed later. In general, the main rule for ready injection of a given carrier is the favorable energy alignment of the contact with the respective carrier band [34] . This rule is obeyed in the cases presented in Fig. 5 , as the alignment of ZnO and TiO 2 CB correspond to the PbS CB, while FTO, Au and PEDOT make a closer contact to the VB. On the other hand, knowledge of metal semiconductor contacts shows additional important mechanisms, for example a heavily doped material as FTO forms a very thin interfacial layer that facilitates tunneling. Another consideration frequently used in p-i-n type solar cells and OLEDs is the doping of the contact layer, as n-type layer preferentially takes electrons and conducts holes, and vice versa for a p-type interfacial layer. However, the type of conductivity does not generally determine the type of contact. One example is MoO 3 , which has a very large work function and is strongly n-type. This semiconductor (not presented herein) aligns with the VB (HOMO) of the organic layers, while the energy difference is taken by an interface dipole. Even though it is n-type, MoO 3 forms a selective contact to holes in organic layers, by electron extraction through the CB of the oxide, which is situated only 0.6–0.7 eV above the HOMO of the organic film [35] . These examples indicate that although general rules are useful for basic understanding of tendencies of data of different materials, interfaces must be separately investigated when the type of injection and energy alignment mechanism needs to be really established. Another essential problem that must be considered is the simultaneous contact of electrons and holes in the case in which carriers are similarly abundant in the photoactive layer, which is the case in the CQD solar cells, in which the QD layer is an ambipolar conductor, and also probably in recently developed nanostructured solar cells with organometal halide perovskite absorbers [36] . To explain the operation of selective contacts, and derive useful parameters, a theory of charge generation and contact equilibration is developed in the following paragraph. 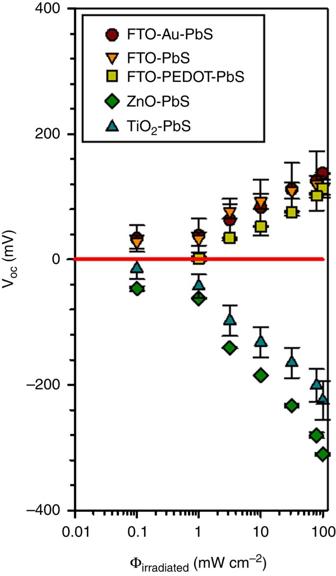Figure 5: Open-circuit potential as a function of light intensity. Evolution of the open-circuit voltageVocwith illumination intensity obtained experimentally for different metal or semiconductor/QD contacts. The open-circuit photovoltage were recorded for an interval of 120 s and plotted Voc and error bars refers to the average value measured and standard deviation respectively. Figure 5: Open-circuit potential as a function of light intensity. Evolution of the open-circuit voltage V oc with illumination intensity obtained experimentally for different metal or semiconductor/QD contacts. The open-circuit photovoltage were recorded for an interval of 120 s and plotted Voc and error bars refers to the average value measured and standard deviation respectively. Full size image Theory of selective contacts in ambipolar materials The model used to explain the experimental results and provide deeper insight into the operation of contacts on photovoltaic CQD films is shown in Fig. 1b . We consider a thin homogeneous quantum dot layer of length L , contacted on the right to a field shielding electrolyte, that penetrates the film up to the substrate layer. This substrate layer, where the CQD film is deposited, forms the left contact. Hereafter we denote such conducting layer the metal contact, although it may be formed by a high-conducting transparent metal oxide covered with additional contact layer as commented in the experimental part. The electronic states in the CQD film are mainly parametrized by the CB and VB levels, more specifically the minimum of the CB edge E c and the maximum of the VB edge E v . These transport states allow fast horizontal equilibration of carrier distributions across the film. In addition, CQDs may have states in the bandgap, such as surface states at the metal–CQD interface at energy E ss . At equilibrium, we have the following equalization of Fermi levels For simplicity, we assume that the QD layer is intrinsic with equilibrium Fermi level E F0 at the center of the gap, to highlight the possibility of shift of both Fermi levels, for electrons and holes. The arguments employed are still valid for doped layers. Establishing equilibrium condition in equation (2) from materials that initially differ in their work function implies that a surface dipole of vacuum level step Δ 0 is formed at the metal contact. When the QD layer is illuminated, electrons and holes are created in the bulk layer at a rate at position x , where α is the absorption coefficient and Φ 0 is the incident photon flux. The creation of excess carriers produces the separation of Fermi levels E Fn and E Fp for electrons and holes, respectively. Carrier densities n and p for the electron and hole densities in CB and VB respectively, are given by the Boltzmann statistics as follows Here k B T is the thermal energy, N c and N v are the effective densities of states at CB and VB, respectively, and n 0 and p 0 the densities taken at equilibrium. In equations (3) and (4), we define separate internal photovoltages of electrons and holes V n and V p , respectively. It should be noted that, as the QD layer is thin, the quasi-Fermi levels of electrons and holes, and therefore V n and V p , are considered uniform over the layer. In this model system, three different kinetic features determine carrier densities and the position of Fermi levels out of equilibrium and consequently V oc . First, band-to-band recombination of electrons and holes. Second, the exchange of carriers between CQDs and the electrolyte. And third, the exchange of electrons and holes at the metal contact, which is the key physical feature that we discuss in this paper. By the first mechanism, the carriers recombine at a rate , where B is a constant, although more generally, but not further mentioned here, recombination may occur via trap states. At the QD–electrolyte contact, both electron transfer with a kinetic constant k cb and hole transfer ( k vb ) can occur, via surface states or via CB/VB, from the quantum dot to acceptor species in solution, or vice versa. At the metal–QD contact, electrons and holes can either transfer from the CB/VB of the QD to the metal Fermi level E Fm , or reciprocally hop from E Fm to CB/VB states or, more generally, first hop to surface states present in the QD bandgap as suggested in Fig. 1b and then from the surface states to the bulk states of the QD. One important aspect of the kinetic exchange at this interface is that it will most probably be dominated by the QD’s that are in direct contact with the metal, as direct tunneling falls off exponentially with distance. Therefore, this transference, either through surface states or to the quantized energy levels of the CB or VB, is considered to occur only to a specific localized system. A well-known model to describe such an exchange is the Marcus model for the transference between a metal and the redox species at the surface [37] . An exchange model between the metal and localized states in the vicinity of the contact has been also widely explored for disordered organic materials that are used in OLEDs [38] , [39] , [40] , [41] . For the present system, as there is a wide variability in the contacts that can be used in solid CQD films, we aim to formulate a theory that can describe carrier exchange without resorting to highly specific details of the contact materials. The main property we wish to describe is the simultaneous presence of electrons and holes at the interface, in which the contact will preferentially pick one kind of carrier to extract. We assume that the variation of voltage is absorbed by the dipole layer Δ at the interface as shown in Fig. 1b . Indeed the role of such dipole layer has been emphasized also in the field of OLEDs. Interfacial dipole layers are used to reduce the effective work function of a metal such as Al (refs 42 , 43 ) and facilitate tuning the energy level of the cathode to the organic material. Dipole considerations have been also recently developed to explain the improved hole injection at the PbS-QD–metal interface at the back contact in CQD solar cells, modified to include an MoO 3 non-stoichiometric interfacial layer [12] . The archetypal model for charge transfer is Butler–Volmer current at the electrochemical interface, that depends on a changing voltage drop at the Helmholtz layer. In our case, however, a voltage difference for either of the two carriers must be formulated in terms of differences of Fermi levels. We therefore suggest the following expressions for the electron current across the interface and similarly for holes The empirical constants β l ( l=n,p ) correspond to the familiar asymmetry factors of the Butler–Volmer model and allow us to satisfy a detailed balance so that equation (2) is recovered in equilibrium. As a particular case, the Miller–Abrahams hopping rate for injection between the metal and the organic corresponds to the case β l =1 in the above expressions. The constants and correspond to the classical role of exchange current and have a main role in establishing the nature of the contact with respect to either electrons or holes equilibration. The explicit dependence of and on the nature of the metal contact implies the knowledge of the interaction between metal and QD across the dipole layer, which is beyond the scope of this work. We refer to the literature for specific models of this type [38] , [39] , [40] . It is readily observed in Fig. 1 that the current extracted from the metal contact is In addition, we can use the continuity equations for electrons and holes, integrating along the QD layer (between 0 and L , and considering a very thin layer), and they give the following results where band-to-band recombination and recombination with the electrolyte have been taken into account. At open-circuit voltage, equation (7) provides the following condition It is obtained from equation (10) that k cb ( n−n 0 )= k vb ( p−p 0 ), or using equations (3) and (4): As shown in the seminal paper by Hodes et al ., [22] preferential charge transfer rates for either electrons or holes to the electrolyte may turn a CQD film into a predominantly n- or p-type semiconductor. In our model however, we assume that transfer rates from the QD layer to the electrolyte are equal in equilibrium, k cb n 0 = k vb p 0 and this implies that V n =V p in all conditions. In this case, the sign of V oc only depends on the kinetic of charge transfer at the contact metal–QD interface, that is, depends on and . In principle, V oc should also depend on β l , however, as mentioned previously, β l has been fixed to unity for the transition at the metal–QD interface. Summarizing, the variation of Fermi levels due to illumination and recombination induces a variation of the metal Fermi level that is absorbed by a correspondent variation of the interfacial dipole at the metal/QDs, so that no band bending occurs at all. The actual variation of the metal Fermi level, in terms of sign and amplitude, that determines V oc , depends on the capability of the interface to more efficiently extract holes or electrons and on the position of the different Fermi levels. From the above equations, we can compute the V oc according to specific assumptions for the contact properties represented by the parameters and β l . We will discuss the influence of the generation/recombination processes at the QDs bulk and at metal/QDs contact on the sign and amplitude of V oc . 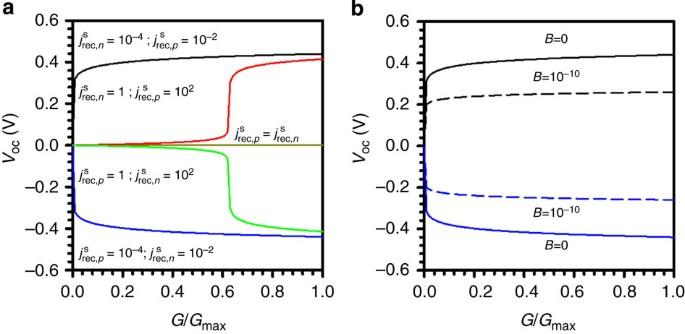Figure 6: Theoretical predictions. Variation of the open-circuit voltageVocwith illumination. (a) Influence of surface recombination at the metal/QDs contact with no bulk recombination (B=0). In this graphic, current densities are expressed in mA cm−2. (b) Influence of the bulk recombination in QDs. The black and blue solid line plots are the same as that given in panela. The dashed line plots correspond to the same respective solid line plots but with a different recombination rate (indicated on the graphic in cm−3s−1units). Other parameters of the simulation:α=105cm−1, Φ0=1017s−1cm−2,d=10 nm,Ec=0.5 eV,Ev=−0.5 eV,Nc=Nv=1020cm−3,kcb=kvb=10 s−1,βn=βp=1. Figure 6a shows the dependence of V oc sign on the ratio / , by a distinction of three cases: (i) > , (ii) < and (iii) = . In the first case, E Fm will tend to equilibrate with E Fn and V oc <0. It should be noted that the higher with respect to , the closer E Fm to E Fn and hence the closer V oc is to its maximum (when V n = V p , V oc(max) = V n = V p ). Inversely, for case (ii), E Fm tends to equilibrate with E Fp and V oc >0. In the end, for symmetrical case (iii), E Fm does not depart from its equilibrium position and V oc =0. Figure 6: Theoretical predictions. Variation of the open-circuit voltage V oc with illumination. ( a ) Influence of surface recombination at the metal/QDs contact with no bulk recombination ( B =0). In this graphic, current densities are expressed in mA cm −2 . ( b ) Influence of the bulk recombination in QDs. The black and blue solid line plots are the same as that given in panel a . The dashed line plots correspond to the same respective solid line plots but with a different recombination rate (indicated on the graphic in cm −3 s −1 units). Other parameters of the simulation: α =10 5 cm −1 , Φ 0 =10 17 s −1 cm −2 , d =10 nm, E c =0.5 eV, E v =−0.5 eV, N c = N v =10 20 cm −3 , k cb = k vb =10 s −1 , β n = β p =1. Full size image We now analyze the influence of the ratios: j s rec / j G and j b rec / j G , as shown by Fig. 6a,b , where j G = qLG and j b rec =qLUnp are the generation and bulk recombination current, respectively, see equations (8) and (9). When > , the metal Fermi level tends to be closer to E Fn than E Fp . However, for a given material under a critical illumination threshold, it is possible that both currents and remain higher than j G ( j s rec ≥ j G ). In this case, the photogenerated carriers directly recombine at the metal–QDs interface and the Fermi levels do not move from their initial equilibrium position. Consequently, before reaching the illumination threshold, we have V oc =|V n |=|V p |=0 (red curve of Fig. 6a ). When j s rec ≤j G , the Fermi levels depart from their equilibrium position and V oc increases. A symmetrical analysis for case ii) can be made, when < (green curve). In Fig. 6b , the influence of the ratio j b rec / j G on the V oc amplitude is also shown. At lower illumination, recombination is lower and therefore, no illumination threshold is observed here. Bulk recombination only affects the maximum value of V oc for a given illumination. In prior reports, it has been generally observed that solar cells based on CQD solids rely on the establishment of a depletion region for the preponderance of photocurrent they extract [2] , [5] . The low fill factor consistently observed in these devices is readily explained by this reliance on a drift in a depletion region, a process that is not normally retained at the device’s maximum power point. We explored herein instead the mechanism in which carriers travel by diffusion, where the recombination lifetime is sufficiently long for the carriers to possess sufficient diffusion length to cross the whole film by hopping from one dot to another one. We found that the sign of V oc depends on the material contacting the CQD PbS films. Under dark conditions, E F of the PbS film is in equilibrium with electrolyte and the metal work function or semiconductor Fermi level of the contact. Under illumination, this equilibrium is broken, and E F in the QDs is split in electron and hole Fermi levels. We developed a theoretical framework for contact equilibration that shows that, depending on the selective contact used, the film produces a preferential charge extraction by the contacts. This model describes well the data in Fig. 5 , where FTO, gold and PEDOT show a positive V oc sign as consequence of preferential hole transfer mechanism, while for ZnO and TiO 2 contacts, a preferential electron transfer mechanism is observed and consequently, negative V oc values. To the best of our knowledge, this work presents first results on the polarity of photovoltage in PbS colloidal QDs solar cells due to electron- and hole-accepting capabilities of selective contacts and highlights the potential of these films in new photovoltaic and optoelectronic devices developed by the kinetic control at contacts. Specifically, our findings indicate that, once minority carrier diffusion lengths are further extended in CQD solids, these materials will be well poised to take advantage of the action of carrier-selective contact engineering. Substrate preparation Different materials were employed as selective contacts. All the studied substrates, which include mesoporous TiO 2 and ZnO electrodes, metallic gold contacts and polymeric PEDOT:PSS films, were deposited over bare fluorine doped tin oxide (FTO). (Pilkington TEC15, ~15 Ω per square resistance), which were previously rinsed with acetone followed by sonication in a mixture isopropanol: water ( v / v =1:1). Before substrates manufacture, precleaned glasses were treated in a UV−O 3 chamber for 5 min. Mesoporous TiO 2 and ZnO electrodes were prepared following the procedures previously reported by Pattantyus-Abraham et al . [30] . For the TiO 2 substrates, the FTO glasses were immersed in a bath of titanium tetrachloride (60 nM in water) at 70 °C for 30 min, and after washing with de-ionized water were heated at 520 °C in a tube furnance for 1 h. This treatment improves the bridging between FTO and TiO 2 nanoparticules. For the nanoparticulated film TiO 2 paste, purchased from Dyesol (18-NRT, particle size=20 nm), diluted ( w / w =1:3) in terpineol was spin-cast at 1,500 r.p.m. for 90 s on the FTO substrates. One edge of the substrate was cleaned with isopropanol to obtain a clean FTO region, which allows electrical contact. TiO 2 films were sintered on a hot plate for 1 h at 400 °C. Finally, the initial TiCl 4 treatment was repeated, in this case to obtain a good electrical contact between the nanoparticles. The thickness of resulting photoelectrodes were ~600 nm determined by profilometry. The preparation of ZnO mesoporous substrates was carried out according to Ip et al . [4] ZnO substrates have been treated with TiCl 4 and likely a TiO 2 was formed in the surface. The metallic gold layer (~60 nm) was deposited on the FTO substrate by a thermal evaporation, where gold was evaporated at a base pressure of 3 × 10 −6 mbar and a rate deposition of 0.04–0.08 nm s −1 . The polymeric poly(3,4-ethylenedioxythiophene) poly(styrenesulfonate) (PEDOT:PSS) substrates were prepared by spin coating in air at 5,500 r.p.m. for 30 s on the FTO substrate. The substrates were heated at 120 °C for 10 min to remove traces of water (film thickness ~35 nm, determined by profilometry). Preparation of the PbS NC film Oleic acid-capped PbS QDs dispersed in octane were synthesized by hydrothermal method as described in previous papers [3] . Multilayered PbS CQD films were deposited under ambient conditions by spin coating following the next steps: (1) 40 μl of oleic-capped QDs (50 mg ml −1 ), (2) 40 μl mercaptopropionic acid ( v / v =1:10) in methanol, (3) rinse with 40 μl of methanol and (4) rinse with 40 μl of octane. The spin coating was performed at 2,500 r.p.m. for 10 s and this protocol was repeated eight times to achieve the desired film thickness. The devices were then stored in nitrogen glove box. Film characterization The optical absorption spectra of the photoanodes were recorded at 600–1,100 nm by a homemade intensified charge-coupled device (ICCD)-based spectrometer. The setup is based on ICCD from Andor (iDUS-420 series) equipped with a grating spectrograph from Oriel (model 77400). A halogen lamp and a set of focusing lenses were used to register the corresponding absorption spectra. Photoelectrochemical characteristics of the device were studied using an FRA-equipped PGSTAT-30 from Autolab and a Keithley 2612 System Source Meter. A three-electrode configuration was used where a Pt wire was connected as counterelectrode and a silver wire as reference electrode. Anhydrous and degassed tetramethylammonium perchlorate (0.1 M) in dimethylformamide was used as non-redox electrolyte. The electrodes were illuminated using a 450 W Xe lamp (Oriel), where the light intensity was adjusted with a thermopile to 100 mW cm −2 , with illumination through the substrate. Cyclic voltametries were recorded at a scan rate of 100 mV s −1 . Measurements were performed from positive to negative potentials for substrates, which are expected to show a preferential hole transfer dynamics (FTO, Au and PEDOT:PSS), and to negative from positive direction for electrodes, which are expected to show a preferential electron transfer dynamics (TiO 2 and ZnO). For the photoinduced open-circuit voltage measurements, the cell was illuminated to a steady voltage. The open-circuit photovoltage were recorded for an interval of 120 s and V oc analysis refers to the average value measured. OCV were recorded at different illumination intensities. The stability of the films has been commented in Supplementary Fig. S1 . How to cite this article: Mora-Sero, I. et al . Selective contacts drive charge extraction in quantum dot solids via asymmetry in carrier transfer kinetics. Nat. Commun. 4:2272 doi: 10.1038/ncomms3272 (2013).